Seismic evidence of a two-layer lithospheric deformation in the Indian Ocean Intra-plate deformation and associated earthquakes are enigmatic features on the Earth. The Wharton Basin in the Indian Ocean is one of the most active intra-plate deformation zones, confirmed by the occurrence of the 2012 great earthquakes (Mw≥8.2). These earthquakes seem to have ruptured the whole lithosphere, but how this deformation is distributed at depth remains unknown. Here we present seismic reflection images that show faults down to 45 km depth. The amplitude of these reflections in the mantle first decreases with depth down to 25 km and then remains constant down to 45 km. The number of faults imaged along the profile and the number of earthquakes as a function of depth show a similar pattern, suggesting that the lithospheric mantle deformation can be divided into two layers: a highly fractured fluid-filled serpentinized upper layer and a pristine brittle lithospheric mantle where great earthquakes initiate and large stress drops occur. The Indian Ocean Basin is one of the most active intra-plate deformation zones on the Earth [1] , [2] , [3] , [4] , [5] . The deformation is due to the differential rate of subduction/collision of the Indo-Australian plate beneath the Eurasia and Sunda plates. The deformation seems to have initiated ∼ 15 Ma ago [6] and was enhanced around 8 Ma ago when the Tibetan plateau attained its maximum elevation [7] . The weak rheology of the Ninety East Ridge (NER) acts as a boundary for strain orientation and deformation style [5] , [8] , [9] , causing different types of deformation in the Central Indian Basin (CIB) and the Wharton Basin (WB). To the west of the NER in the CIB, deformation is taking place along E-W trending high-angle thrust faults and associated folds [1] , [2] , [3] due to the N-S compression resulting from the continental collision of India with Eurasia. To the east of the NER in the WB, the direction of the maximum stress is NW-SE, and the deformation is accommodated along N5°E-trending re-activated fracture zones with left-lateral strike-slip movements [2] , [5] , [10] , [11] . This was recently confirmed by the occurrence of the Mw=8.6 earthquake on April 11, 2012 in the WB, the largest strike-slip earthquake ever observed on the Earth. It was preceded by a foreshock of Mw=7.2 on January 10, 2012 and followed by an aftershock of Mw=8.2 (ref. 12 ) along with many small aftershocks, suggesting that the WB is indeed deforming actively. The lithosphere in the WB was created at the Wharton Spreading Centre (WSC) between 133 and 40 Ma ago [13] , [14] . A major reorganization of the Indian Ocean ridge system occurred following the initial collision of India with Eurasia ∼ 50 Ma ago and the cessation of spreading at the WSC around 40 Ma ago, after which India and Australia became a single plate. Present-day intra-plate left-lateral deformation in the WB is consistent with the increasing obliquity and decreasing convergence rate of the Indo-Australian plate from Java (orthogonal at 60 mm yr −1 ) in the east to Sumatra (54 mm yr −1 ) in the west, and nearly arc-parallel near the Andaman Islands (43 mm yr −1 ) [15] . Based on bathymetry and shallow seismic data, Deplus et al . [5] suggested that the differential motion in the WB is accommodated along re-activated N5°E trending fracture zones although NE-SW lineation gravity indicates some folding [5] , [16] . Most of the earthquakes in the WB have left-lateral strike-slip motion, with a few earthquakes having normal or thrust motions ( Fig. 1 ). Based on waveform analyses, Robinson et al . [17] suggested that the 2000 Mw=7.9 Cocos earthquake did not only rupture a re-activated N5°E fracture zone but possibly also an orthogonal E-W trending ridge parallel fault. Some active thrust faults are also reported with an orientation perpendicular to the NW-SE compressive axis [10] . The 10 January foreshock (Mw=7.2) and 11 April aftershock (Mw=8.2) seem to have ruptured the re-activated fracture F6 ( Fig. 1 ), but the slip during the Mw=8.6 earthquake is more complex, involving several near-orthogonal fault segments [12] , [18] , [19] . While some authors argue that only the NNE-SSW fault plane along a fracture zone (F6) ( Fig. 1 ) was re-activated [20] , some others suggest that new lithospheric faults, not the existing fabric, were initiated [18] . 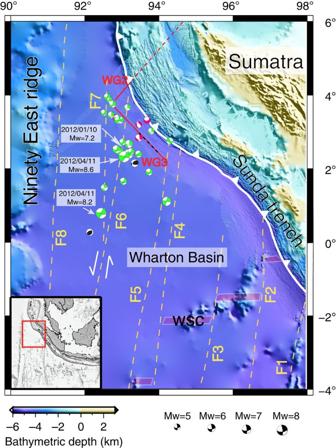Figure 1: Study Area. The red lines indicate the seismic profiles WG3 and WG2, with solid lines showing the part of the profiles used in this study. The black dashed line indicates the portion of the seismic image shown inFig. 4. Yellow dashed lines indicate the fracture zones marked by F1-F8. WSC: Wharton Spreading Centre. The beach balls indicate earthquakes with Mw≥4.8 that have a CMT solution in the area where the lithosphere is∼56 to 60 Ma old (seeTable 2). Normal: Red, Strike-slip: Green, Thrust: Black. The red rectangle in the insert indicates the location of the study area. The locations of the three 2012 earthquakes discussed in the text are also marked. Figure 1: Study Area. The red lines indicate the seismic profiles WG3 and WG2, with solid lines showing the part of the profiles used in this study. The black dashed line indicates the portion of the seismic image shown in Fig. 4 . Yellow dashed lines indicate the fracture zones marked by F1-F8. WSC: Wharton Spreading Centre. 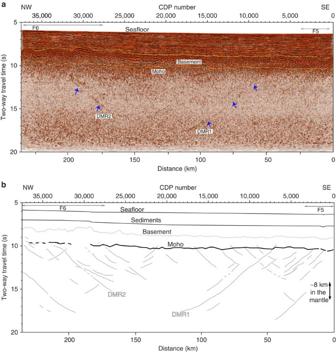Figure 2: Time Seismic image and interpreted faults. (a) Post-stack time domain migrated seismic reflection image along profile WG3. F5 and F6 indicate the crossing of the fracture zones. DMR1 and DMR2 are the deep mantle reflectors. (b) Line drawing of interpreted reflections from the migrated section shown ina. The beach balls indicate earthquakes with Mw≥4.8 that have a CMT solution in the area where the lithosphere is ∼ 56 to 60 Ma old (see Table 2 ). Normal: Red, Strike-slip: Green, Thrust: Black. The red rectangle in the insert indicates the location of the study area. The locations of the three 2012 earthquakes discussed in the text are also marked. Full size image A marine seismic survey was conducted offshore northern Sumatra in 2006 to investigate the structural properties of the Sumatra subduction zone [21] . Our study area is located ∼ 100 km north of the 2012 main shock, close to the 10 January foreshock. We focus on a 233-km-long trench-parallel seismic profile (WG3) and a small segment of the orthogonal profile WG2 ( Fig. 1 ). Profile WG3 runs between 32 and 66 km from the subduction front over a 55–58 Ma old oceanic crust [22] ( Fig. 1 ). Using these data, we describe the shallow deformation and their link with deep mantle faults, and shed light upon the nature of the lithospheric deformation in the WB. The seismic image shows dipping reflections down to 45 km depth, which we interpret as deep penetrating mantle faults. The number of faults first decreases with depth down to 25–30 km and then remains constant down to 45 km depth. The relative amplitudes of these reflections also first decrease with depth down to 25 km and then remain constant down to the base of the lithosphere. A similar behaviour is observed for a number of earthquakes originating in the mantle. These results suggest that the deformation in the mantle consists of two layers, an upper serpentinite layer (SL) where a large number of earthquakes occur and a pristine layer (PL) where great earthquakes initiate and large stress drops occur. The boundary between the SL and PL is likely to be responsible for the presence of the double Bennioff Zone observed in subudction zones worldwide. Shallow structures The deep seismic reflection profile WG3 crosses the northern extremity of one of the fault segments of the 2012 Mw 8.6 WB intra-plate strike-slip earthquake. The entire WG3 seismic image in the two-way-travel time domain is shown in Fig. 2a and its interpreted line drawing is shown in Fig. 2b . We depth converted the seismic image ( Supplementary Fig. 1 ) using a one-dimensional velocity ( Supplementary Fig. 2 ) determined from a combination of seismic tomography acquired along an orthogonal profile [23] and mantle velocity determined for oceanic mantle formed at the fast spreading East Pacific Rise [24] . The details of the data acquisition and processing can be found in the Methods section. The water depth varies from 4.7 km in the southeast to 4.4 km in the northwest whereas the sediment thickness decreases from 3.5–4 km to 2.5–3 km ( Supplementary Fig. 1 ). Most of the sediments are recent, supplied from the Nicobar fan over the last 15 Ma, and record recent tectonic history. The top of the oceanic crust and the oceanic Moho are well imaged along most of the profile ( Fig. 2 , Supplementary Fig. 1 ). The crust in this area is thin, possibly due to the ridge-plume interaction [22] . The ridge-plume interaction usually tends to produce a thicker crust, but it can also lead to the formation of thinner crust due to the formation of cold channels around plumes [25] , [26] and their interaction with a spreading centre. Figure 2: Time Seismic image and interpreted faults. ( a ) Post-stack time domain migrated seismic reflection image along profile WG3. F5 and F6 indicate the crossing of the fracture zones. DMR1 and DMR2 are the deep mantle reflectors. ( b ) Line drawing of interpreted reflections from the migrated section shown in a . Full size image The profile crosses two fracture zones, F5 and F6: F5 can be identified by a depression on the seafloor and in the basement near CDP 1500 in the SE, and F6 by a ∼ 60-km wide complex basement high starting from CDP 29000 to the end of the profile in the NW [27] ( Fig. 3 ). The faults in the sediments reaching up to the seafloor suggest that both F5 and F6 have been re-activated in the recent past. The narrow zone (2 km) of deformation at F5 indicates the existence of strike-slip faulting. The deformation along F6 is characterized by several eastward-dipping faults. The dip of these faults is steep, between 50° and 75°. Bathymetry data suggest that the strike of these faults is N-S, parallel to the strike of F6 (ref. 27 ), suggesting the re-activation of F6 in a very broad zone. The top of the oceanic crust between F6 and F7 is dominated by complex topography ( ∼ 2 km wide and ∼ 1 km high), indicating that this region is geologically complex, as indicated by the magnetic anomaly study [28] and orthogonal seismic profile [27] . In between these two fracture zones, only lower sedimentary strata are deformed and faults initiate from the basement but do not reach the seafloor, implying that the deformation between the fracture zones ceased some time ago and most of the motion might be accommodated along these fracture zones. Since our profile is parallel to the subduction front, it would be difficult to image trench-ward dipping normal faults in the sediments, but the dip-slip motion observed over F6 might be due to bending related stress [27] . 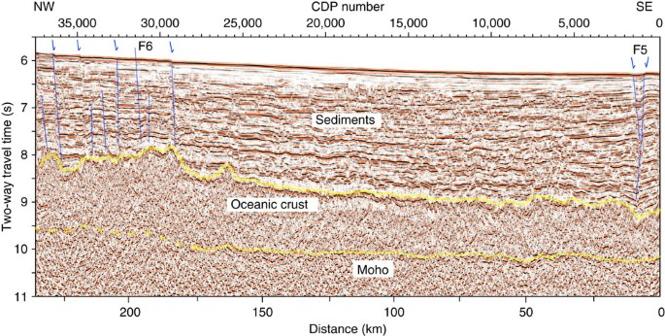Figure 3: Shallow part of WG3 seismic reflection image. The interpreted seismic reflection image along WG3 in the time domain. The faults in the region of the two fracture zones F5 and F6 are marked by blue lines and arrows. Yellow lines highlight the oceanic crust and the Moho. Figure 3: Shallow part of WG3 seismic reflection image. The interpreted seismic reflection image along WG3 in the time domain. The faults in the region of the two fracture zones F5 and F6 are marked by blue lines and arrows. Yellow lines highlight the oceanic crust and the Moho. Full size image Mantle reflections The most striking feature in this seismic image is the presence of a large number of dipping reflectors in the mantle ( Supplementary Fig. 3 ); one of them penetrates down to 45 km depth (DMR1), the deepest reflection ever imaged within the oceanic lithosphere ( Fig. 4 ), and a second one (DMR2) extends down to 37 km. These reflections are real and are not associated with scattering effects from the seafloor or the basement [27] . A pre-processed super common mid-point gather clearly shows the reflector event corresponding to the DMR1 at 17.25 s ( Fig. 5 ). Although some dipping reflections are present in the crust ( Supplementary Fig. 4 ), the dipping mantle reflections are seldom seen cutting through the crust; rather they tend to initiate near the Moho and continue down into the mantle until at least 20–30 km, some of them up to 45 km. The relationship between these deep reflectors and shallow deformation is unclear, as we do not observe any continuous events connecting the faults imaged in the sediments with the deep reflectors through the crust. The dip of these mantle reflections is between 25° to 35°, and they dip in both directions. Although profile WG3 is not orthogonal to the oceanic fabric (E-W spreading and N-S fracture zones), we can project the two major faults (DMR1 and DMR2) to different strikes. We find that the dip of these reflections only increases to 30–45° (see Methods, Supplementary Figs 5 and 6 ). 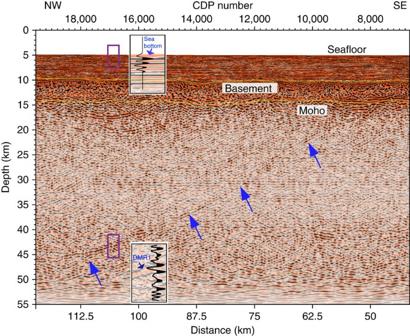Figure 4: Seismic reflection image of the deepest fault (DMR1). The arrows mark the position of the deep penetrating fault. The purple rectangles indicate the blow-up of seismic images and wiggle traces of the seafloor and the deep mantle reflector shown adjacent to them. An automatic gain control with a 3 km-long window was applied to enhance the reflections at depth. For precise location of the image seeSupplementary Fig. 1. Figure 4: Seismic reflection image of the deepest fault (DMR1). The arrows mark the position of the deep penetrating fault. The purple rectangles indicate the blow-up of seismic images and wiggle traces of the seafloor and the deep mantle reflector shown adjacent to them. An automatic gain control with a 3 km-long window was applied to enhance the reflections at depth. For precise location of the image see Supplementary Fig. 1 . 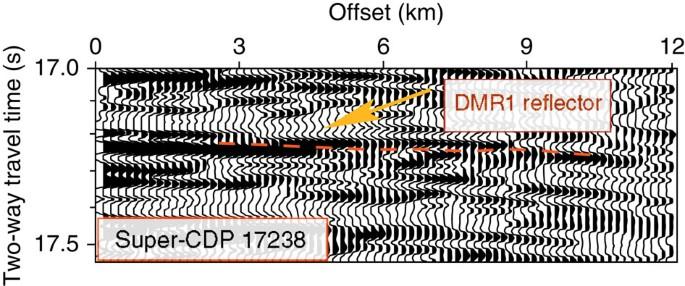Figure 5: Super-CDP gather. Super-CDP gather 17283 showing DMR1 reflector as a function of offset at 17.25 s. Full size image Figure 5: Super-CDP gather. Super-CDP gather 17283 showing DMR1 reflector as a function of offset at 17.25 s. Full size image We estimated the polarities of deep reflections and of the seafloor by summing dozens of migrated traces on the seafloor and at different depths along the deep reflections. The results show that the polarity of the DMR1 is reverse to that of the seafloor ( Fig. 4 ). Since the velocity increases with depth below the seafloor, the medium in the immediate vicinity of the reflector should have a lower velocity when compared to that of the surrounding bulk medium. Thus the negative polarities suggest that the deep reflections are produced by negative velocity (impedance) contrasts. The dominant frequency of these reflections is 7–10 Hz ( Supplementary Fig. 7 ), hence the dominant wavelength would be ∼ 1 km for a mantle P-wave velocity of 8 km s −1 , therefore the thickness of the reflective zone has to be at least 250–1,000 m in order to be imaged by a seismic method. In order to gain more insight on these deep reflections, we show seismic images along profile WG3 and an orthogonal profile WG2 ( Fig. 1 ), using a 3D perspective view ( Fig. 6 ). The crustal features on the WG2 profile are similar to those observed on WG3, but a fault is seen to cut through the entire crust and connects with a fault in the sedimentary layer at the top and with a mantle reflector near the bottom, showing that crustal faults can be imaged if they are shallow dipping. 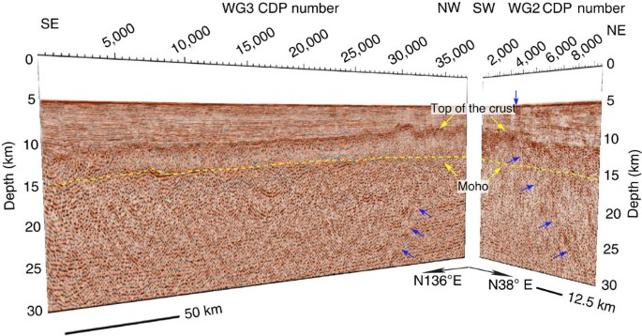Figure 6: 3D view of seismic images along profiles WG2 and WG3. The oceanic part of WG2 profile (right) and the whole WG3 profile (left) in the depth domain. Blue arrows mark dipping reflections. Both profiles cross fracture zone F6. A trench-ward dipping reflection can be followed from the seafloor down to 30 km depth. Figure 6: 3D view of seismic images along profiles WG2 and WG3. The oceanic part of WG2 profile (right) and the whole WG3 profile (left) in the depth domain. Blue arrows mark dipping reflections. Both profiles cross fracture zone F6. A trench-ward dipping reflection can be followed from the seafloor down to 30 km depth. 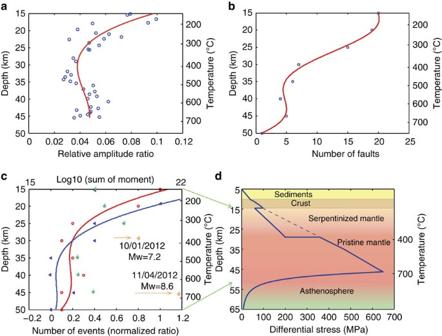Figure 7: Depth dependent parameters. (a) Relative amplitude ratio of the mantle reflector (DMR1) as a function of depth/temperature. The amplitude has been compensated for geometrical spreading and attenuation (Qp=1,000). The blue circles are the ratio of amplitudes (see Methods) and the red curve is a fitted curve using a 3rd order polynomial. (b) Number of faults observed along 233-km-long seismic profile WG3 inFig. 2bas a function of depth/temperature. The numbers of faults are estimated by drawing a horizontal line across the whole section at 5 km interval and counting the number of intersecting faults (Table 1). Blue circles represent the number of faults picked in a 5 km vertical bin. The red curve is a 4th order polynomial fit. (c) The number of earthquakes and their cumulative moments as a function of depth/temperature for oceanic lithosphere of 50–60 Ma. Circles and red curve are local earthquakes shown inFig. 1while triangles and blue curves are global data and their fits30. Both data have been normalized separately and the number of events is in a 5 km depth bin. Green stars are the cumulative moments of the local earthquakes inTable 2in the 5 km depth bin. The moments of the Mw=7.2 and Mw=8.6 2012 earthquakes (orange stars) stand out. (d) The approximate differential stress as a function of depth/temperature for a 60 Ma lithosphere. Dash blue line represents the Byerlee law for a normal lithosphere of 60 Ma. Full size image Depth dependence Figure 7a and Supplementary Fig. 8 show the ratio of amplitudes of the two main dipping reflections (DMR1, DMR2) and the seafloor reflection as a function of depth and temperature. The ratio is ∼ 0.1 just below the Moho at 15 km depth and decreases linearly with depth to a value of ∼ 0.04 down to 25 km. Below this depth, the ratio remains constant at ∼ 0.04 ( Fig. 7a ) down to the 45 km depth. Figure 7b shows the number of reflectors imaged along the profile in the mantle as a function of depth (temperature). We were able to identify 20 dipping reflectors just below the Moho; the number decreases to 7 at 30 km depth and then remains nearly constant at 5 down to 45 km depth ( Table 1 , Fig. 2b ). Figure 7c shows the number of intra-plate oceanic earthquakes as a function of depth for a lithosphere of 50–60 Ma of age, both for local earthquakes in the Wharton Basin [27] , [29] ( Fig. 1 , Table 2 ) and global events [30] . The depth of the global events are well constrained by waveform modelling [30] . For local events, we used re-located events until October 2007 (ref. 29 ) and the GCMT depth for the recent events [27] . Although there could be uncertainties in the depth of these events, they provide a good indication of the pattern of seismicity with depth [31] . We also show the cumulative moment as a function of depth for the local events. These plots clearly indicate that the number of earthquakes linearly decreases down to 25 km and then remains constant below this depth down to 50 km. The cumulative moment increases linearly with depth down to 25 km, then decreases down to 35 km, and then remains constant below this depth, following the pattern similar to the number of faults imaged ( Fig. 7b ). Interestingly, the Mw=7.2 foreshock and Mw=8.6 2012 main shock stand out, having exceptionally large moment, and initiating in the lower part of the lithosphere ( Fig. 7c ). Figure 7: Depth dependent parameters. ( a ) Relative amplitude ratio of the mantle reflector (DMR1) as a function of depth/temperature. The amplitude has been compensated for geometrical spreading and attenuation (Qp=1,000). The blue circles are the ratio of amplitudes (see Methods) and the red curve is a fitted curve using a 3rd order polynomial. ( b ) Number of faults observed along 233-km-long seismic profile WG3 in Fig. 2b as a function of depth/temperature. The numbers of faults are estimated by drawing a horizontal line across the whole section at 5 km interval and counting the number of intersecting faults ( Table 1 ). Blue circles represent the number of faults picked in a 5 km vertical bin. The red curve is a 4th order polynomial fit. ( c ) The number of earthquakes and their cumulative moments as a function of depth/temperature for oceanic lithosphere of 50–60 Ma. Circles and red curve are local earthquakes shown in Fig. 1 while triangles and blue curves are global data and their fits [30] . Both data have been normalized separately and the number of events is in a 5 km depth bin. Green stars are the cumulative moments of the local earthquakes in Table 2 in the 5 km depth bin. The moments of the Mw=7.2 and Mw=8.6 2012 earthquakes (orange stars) stand out. ( d ) The approximate differential stress as a function of depth/temperature for a 60 Ma lithosphere. Dash blue line represents the Byerlee law for a normal lithosphere of 60 Ma. Full size image Table 1 Number of Faults along profile WG3. Full size table Table 2 Earthquakes in the Wharton Basin. Full size table The most important observation from our study is that there are a large number of dipping mantle reflectors imaged in the study area. There are two prominent reflections, DMR1 and DMR2, extending down to 45 and 37 km respectively and dipping in opposite directions. These reflections are rarely imaged going through the crust, although some of them do connect with faults imaged in the sediments. It is possible that the reflectors in the crust are steeply dipping, similar to the faults in the sediments around F6, and therefore, it would be difficult to image them on a trench parallel profile. This is because a steeply dipping fault will offset sedimentary layers vertically, which is easy to identify, whereas a steeply fault in basaltic crust would have the same material on either side of the fault and hence would be difficult to image. The presence of a crustal fault penetrating down to 30 km along profile WG2 further supports this interpretation. This means that the deep mantle faults might be connected to faults observed in the sediments. These reflections could be due to lithospheric faulting, magmatic or thermal cracking processes. The presence of frozen gabbroic melt in the mantle could produce appropriate impedance contrast to generate the observed reflections. The crust in the vicinity of profile WG3 was formed ∼ 56 Ma ago in a fast spreading environment [22] , therefore the mantle must have been hot and the melt mobile, and hence it would have been difficult to retain melt in a steeply dipping narrow zone from the Moho down to 45 km depth; moreover, the maximum dip of imaged crustal magma chamber is 10–15°(ref. 32 ). On the other hand, the thermal stress in-between the fracture zones is strong enough to generate a deep cracking, which could fracture the lithosphere down to ∼ 20 km for a lithosphere of 50 Ma (ref. 33 ). Since the most likely thermal crack system would have a cascade structure composed of widely spaced deep cracks and narrowly spaced shallow cracks [33] , whose dip would be nearly vertical -- much steeper than the mantle reflector imaged in our profile -- these reflectors could not be due to the thermal cracking, and consequently we suggest that these reflections were produced by faulting. There were three strike-slip earthquakes in the WB in 2012, including the Mw 8.6 great earthquake. The Mw 8.6 event was 100 km south of profile WG3 and has a slip down to ∼ 45 km depth on the NNE-SSW trending plane around F6 extending up to profile WG3 (refs 12 , 34 ), and therefore, it is tempting to suggest that this earthquake might have re-activated the DMR2, which also seems to initiate below F6 and extends down to 37 km depth. However, the dip of DMR2 is too shallow (30–40°) as compared to the dips of the 2012 WB earthquakes (>70°), suggesting that DMR2 could not have ruptured during the 2012 strike-slip earthquake. The second major fault DMR1, although extending deeper down to 45 km, lies 105 km eastward of the Mw 8.6 event, also has smaller dip angle, hence could not have ruptured during the great earthquake either. Since the Mw 8.6 great strike-slip earthquake had a very complex fault orientation, it is possible these the faults imaged along our profile might have played some role in this complex faulting mechanism. There are several mechanisms to generate these mantle faults. One possibility is that these faults are generated due to bending-related faulting in the outer rise region. In subduction zones, the incoming plate bends down towards the trench in response to compressive stresses induced at the plate interface, leading to varying degrees of shallow normal faulting and deeper thrust faulting in the outer rise region of the incoming plate [35] , [36] . Although bending related seismicity is termed as ‘outer rise’ earthquakes, most of the earthquakes occur in outer trench slope where the plate curvature is highest, which is generally about 50–75 km seaward off the trench axis [37] . Our profile WG3 lies within 32 and 66 km off the trench, hence in the zone of maximum curvature. Therefore, it is possible that the faults we imaged are related to plate bending. In the Middle American Trench, some of these bending related normal faults have been imaged down to 5–8 km below the Moho [38] . However, the plate bending tends to generate a double stress layer with in-plate tension in the upper layer and in-plate compression in the lower layer [39] , which could produce both a family of normal faults in the upper part and thrust faults in the deeper part with an aseismic zone separating the two types of faulting. The precise depth of the double-stress layer transition zone and its thickness vary depending upon the age of the subducting lithosphere, convergence rate and the dip of the subducting plate [36] . For the northern Sumatra suduction, the normal faulting should extend down to 20–25 km depth, followed by a 5–8 km thick different stress-state layers transition zone, and then thrust faulting should extend down to 50 km depth. However, the deepest reflector imaged on our profile extends from the Moho down to 45 km continuously, without any aseismic gap. Since the pole of plate rotation lies in the diffuse boundary, which includes our study area [40] , the intra-plate stress could get modified, affecting the resulting state of stress in the region and leading to the faulting pattern we observe along our profile. There are only very few normal and thrust earthquakes, most of the earthquakes on the oceanic plate have dominantly strike-slip focal mechanisms ( Fig. 1 ). The thrust events observed after the 2004 earthquake at the subduction front were attributed to a strong coupling between the subducting plate and the overriding plate up to the subduction front, and consequently the seaward propagation of the megathrust rupture up to the trench [21] , [23] . The bathymetry and seismic reflection data indicate that most of the dip-slip faults along F6 and F7 have N-S strike, not trench parallel as expected for bending related faulting. It is possible that the lateral variation in bending related stress due to the curvature at the trench resulting from the obliquity of the subduction, combined with dominant strike-slip deformation pattern in the WB, leads to the complex faulting pattern observed in the region. Besides the plate bending effect in the outer rise, another possibility is that these faults were formed by the reactivation of ridge-parallel normal faults as thrust faults a long time ago and they are inactive now [27] . In the CIB, extensive thrust faults have been imaged cutting through the crust, some of them extending into the mantle [41] , [42] , which are suggested to be due to the active intra-plate deformation in the CIB. There too, not all the mantle faults extend into the crust and subsequently to the sediments, indicating that these faults are either older or associated with the original oceanic fabric. The timing of the faulting would be difficult to estimate, but they must have been formed after several tens of million years from the time of the formation of the oceanic crust for the brittle lithosphere to be thick enough (40–50 km) and to lie below 750 °C (ref. 43 ). The main tectonic events effecting this lithosphere were the collision of India with Australia at ∼ 40 Ma, and the initiation of the deformation in the Central Indian Basin ∼ 15 Ma ago [6] with enhanced deformation at 8 Ma [7] , hence these faults might have been formed during any of these two events. On the other hand, some studies found that the Mw=8.6 event also ruptured NWN-SES faults [12] , [18] , which are unrelated to the oceanic fabric. On the contrary, a recent bathymetric and seismic study indicates the absence of any such WNW-ESE-trending faults [44] . This study also indicates the presence a complex set of Riedel faults with NNE and SSE orientation. It is difficult to distinguish the different origins of these mantle reflections, but the bending related stresses combined with the stresses caused by diffuse deformation in the WB are the most likely cause of these faulting. However, their depth dependent properties provide important insight about the nature of the deformation as a function of depth. The linear decrease in the amplitude ratio of the reflectors with depth cannot be attributed to a temperature-related intrinsic attenuation, because if it were the case, the reflection coefficient should continue to decrease with depth below 25 km. The frequency versus depth plot ( Supplementary Fig. 7 ) indicates that the dominant frequency of DMR1 decreases from 10 to 7 Hz, and hence the effect of the intrinsic attenuation should be small. Assuming a thermal profile for a ∼ 60 Ma old oceanic lithosphere (see Methods), the mantle temperature should be ∼ 150 °C below the Moho increasing to 680 °C at 45 km depth, and hence the attenuation should increase with depth, instead of decreasing, which indicates that the amplitude ratio represents the change in the reflection coefficient (see Methods). The negative polarity of the dipping reflection ( Fig. 4 ) suggests that it should be due to the presence of a thin low velocity zone associated with a fault. The water penetrating along the damaged fault zone, produced by any of the processes discussed above, could serpentinize the mantle peridotite and produce a low velocity reflective zone relative to the surrounding unaltered lithosphere. The serpentinization has also been invoked to explain high heat flow and sub-Moho reflections in the CIB [42] . We used the amplitude ratio to estimate the reflection coefficient of the fault (see Methods), which will depend on its overall degree of serpentinization. A linear decrease in the degree of serpentinization, suggested by the variation in the reflection coefficient between the Moho and the ∼ 25 km depth, may be expected if the pressure promotes the closure of cracks and a reduction of permeability with depth that inhibits fluid circulation and therefore serpentinization. The change in the reflection coefficient at ∼ 25 km depth is associated with a lithospheric temperature of 300–350 °C, which is close to the upper limit of the stability of lizardite serpentinite [45] . The temperature at 45 km depth would be ∼ 680 °C, which is much higher than the stability limit of serpentine at ∼ 400 °C (ref. 46 ). It is interesting to note that the change in the above properties coincides with the aseismic zone at 25–30 km depth that would separate the regions of outer rise bending-related normal faulting from deeper thrust faulting, and would likely inhibit the penetration of fluids into the deeper parts of the mantle [31] . So below 25 km depth, the reflections display a lower velocity contrast that may be due to the presence of other alteration phases, such as antigorite serpentinite that is stable at higher temperature (up to 600–650 °C) (ref. 47 ) or some other processes, such as shear zones. Mylonite shear zones are formed due to the deformation along a fault zone at higher temperatures. The critical temperature over which the ductile deformation predominates is estimated to be 620 (±120) °C for olivine [48] . The brittle-ductile interface would be reached at a depth of 38±8 km for a 60 Ma old oceanic lithosphere [49] . Some peridotite shear zones reach extremely high temperature (600–800 °C), sufficient to form veins of melt that rapidly cool and are chilled to glass [50] , [51] . So at such great depths as DMR1 with high pressure, high temperature and high slip (large magnitude and stress drop caused by great earthquakes, such as the 2004 Sumatra earthquake), the lithospheric failure zone may melt and produce shear zones. The presence of a large number of faults just below the Moho in both WG3 and WG2 ( Figs 2 , 6 and 7b ) extending down to a depth of ∼ 25 km suggests that the upper mantle is extremely fractured. The observation of a large number of earthquakes just below the Moho also supports the idea of a highly fractured upper mantle. The decrease in both the number of faults and the number of earthquakes with depth suggests that deformation decreases with depth down to 25–30 km, which might be associated with the decrease in serpentinization with the increase of temperature. Below 25–30 km, both the number of faults and the number of earthquakes remain constant down to 50 km depth, suggesting a change in the regime of the lithospheric deformation, possibly affected by and also controlling the rheology of the mantle. Figure 7d shows a schematic diagram demonstrating the rheology as a function of depth (temperature). Sediments and the crust follow the Byerlee law rheology [43] . Just below the Moho, the presence of only ∼ 10–15% of lizardite serpentinization can reduce the strength of the lithosphere significantly [52] , and particularly that of serpentinite-bearing faults, owing to its low coefficient of friction relative to the Byerlee law (μ ∼ 0.3–0.4 versus μ ∼ 0.85). At a depth of 25–30 km, at the stability limit of lizardite serpentinite, the strength of the lithosphere should increase due to the change in friction according to the Byerlee law (μ ∼ 0.85). In this case, the result is a strength envelope with a ‘very weak upper mantle’ between the Moho and ∼ 25 km depth and a strong lower mantle down to the base of the lithosphere. This strength envelope is consistent with the seismic moment as a function of depth during the 2012 Wharton Basin earthquakes [12] . Our results suggest that the deformation in the Wharton Basin oceanic lithosphere can be divided into two layers: (i) serpentinized upper lithosphere (SL) from the Moho down to 25–30 km and (ii) a pristine lithospheric mantle (PL) from 25 km down to the base of the lithosphere at 60 km depth ( Fig. 8 ). The finite fault model of the 2012 great Wharton Basin earthquakes also shows two zones of maximum slip, 5–25 km and 30–50 km (ref. 12 ), supporting our idea of a two-layer model of the lithospheric mantle deformation. Numerical modelling studies suggest that the large earthquakes initiate in a large stress-drop regime at greater depth whereas small earthquakes initiate at shallow depth [52] , confirmed by the 2012 earthquakes, supporting our observation. 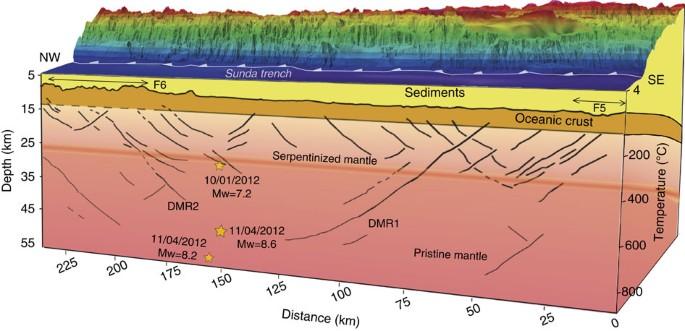Figure 8: Schematic diagram. A 3D block diagram showing the interpreted faults imaged on profile WG3, location of the fracture zones F5 and F6, and projected hypocentres of January and April 2012 earthquakes. The Sunda trench and accretionary prism are also shown in the background. Figure 8: Schematic diagram. A 3D block diagram showing the interpreted faults imaged on profile WG3, location of the fracture zones F5 and F6, and projected hypocentres of January and April 2012 earthquakes. The Sunda trench and accretionary prism are also shown in the background. Full size image Most of the normal earthquakes in the outer arc rise occur in the SL whereas the thrust events initiate below 25 km depth down to 40 km depth [30] in the PL; the deep lithospheric faults imaged here may act as weak zones that may be reactivated as thrust faults. Highly fractured SL should be able to transport a large amount of water in the Benioff zone as suggested by other seismological studies [53] , [54] . The dehydration of serpentinite at the SL/PL boundary may create a reaction zone leading to seismicity and would be helpful to explain the location of the second (lower) Benioff zone observed here in the double Benioff zones (DBZ) [55] , [56] . The thickness of SL/PL will depend on the age of the lithosphere. The subducting slab in our study area contains a ∼ 15–17 km thick SL ( Fig. 7 ), which corresponds to the estimated separation of the Benioff zone for a 56 Ma old lithosphere [56] , and is in an agreement with the observed results offshore Sumatra [56] . We projected earthquake events [57] along a cross section perpendicular to the subduction around WG3 ( Fig. 9a ) to obtain a vertical profile of all the events ( Fig. 9b ), which shows a separation depth of DBZ at 12 ∼ 18 km below the top of the crust ( Fig. 9c ), consistent with the theoretical prediction. A vertical aseismic zone with a thickness of 5 ∼ 7 km separating shallow normal-faulting earthquakes and deeper thrust-faulting earthquakes is also consistent with the double-stress layer paralleling to the Benioff zone in the Sumatra subducting plate [57] . Therefore, the SL/PL boundary observed in our seismic image corresponds to a rheological and alteration boundary that could indeed be the locus of seismicity corresponding to the second Benioff zone. 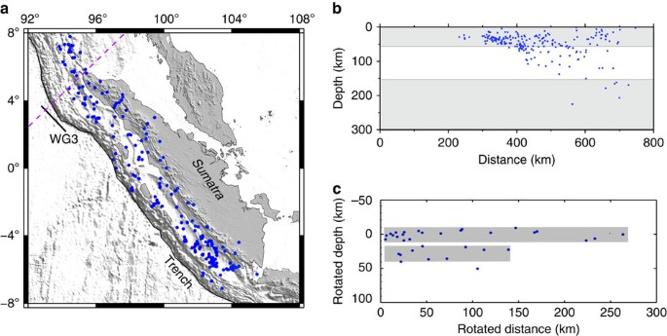Figure 9: Double Benioff Zone. (a) The earthquakes in Sumatra area57. (b) Projected events along a cross section marked by the dashed line inawhich is perpendicular to WG3. The events in the middle white window are used inc. (c) The events versus depth plot showing the Double Benioff Zone. The earthquakes shown in white window inbwere projected at the slab-normal locations and were rotated along the plate interface. Figure 9: Double Benioff Zone. ( a ) The earthquakes in Sumatra area [57] . ( b ) Projected events along a cross section marked by the dashed line in a which is perpendicular to WG3. The events in the middle white window are used in c . ( c ) The events versus depth plot showing the Double Benioff Zone. The earthquakes shown in white window in b were projected at the slab-normal locations and were rotated along the plate interface. Full size image Although our two-layer deformation model explains all the existing seismic and seismological observations, more ultra-deep seismic reflection data from another part of the WB and the CIB are required to quantify the lateral extent of the mantle deformation in the Indian Ocean. Imaging of the crustal faults is also extremely important because of the links between the deep reflectors and the crustal faults are of fundamental importance. The study should be further extended to other outer rise areas using ultra-long streamers to characterise the deformation between shallow normal faulting and deep thrust faulting. Seismic data acquisition The 233-km-long offset deep seismic reflection profile WG3 was acquired by the WesternGeco marine seismic vessel Geco Searcher in July 2006. The profile was shot in a NW-SE direction, nearly parallel to the trench at 32–66 km distance. It covers the entire segment of the oceanic crust, bounded by two fracture zones, F5 and F6 that lie at the southeast and northwest ends of the profile, respectively. WG2 was shot traversing the subduction zone orthogonally with a direction of N38°E crossing the whole subduction system [21] , [58] . Here we only show the oceanic part of the profile ( Fig. 1 ). To enhance low frequency signals, the seismic data were acquired using a 12-km-long streamer towed at 15 m depth. The seismic source was composed of 6 sub-arrays with 8 airguns in each sub-array making a total array volume of 10170 in ref. 3 , with an operating pressure of 2,000 p.s.i. The seismic source was towed at a depth of 15 m and the shot interval was 50 m. The individual hydrophone spacing in the Q-Marine streamer was 3.125 m. After applying digital noise attenuation and appropriate digital spatial anti-alias filters [59] , the digital signals were spatially resampled to 958 channels with a digital hydrophone group interval of 12.5 m. The seismic data record length was 20.48 s with a temporal sample interval of 2 ms. The data were rich in low frequency signal and were very helpful in imaging the deeper structure such as the deep crust and uppermost mantle. Low frequency enhancement In order to image deep structures, one requires low frequency seismic energy as low frequency signals penetrate deeper in the earth due to low attenuation. High frequency energy gets attenuated rapidly with depth. As discussed above, both the airgun source and the streamer were deployed at 15 m water depth. Since the sea surface acts like a mirror, with a reflection coefficient of −1, it reflects both the seismic source energy at its generation ( Supplementary Fig. 9b ) and the up propagating seismic wavelet at the receivers ( Supplementary Fig. 9c ) during recording, and produces almost perfect reflections as well as a phase change as shown in Supplementary Fig. 9e ; these are called ghosts ( Supplementary Fig. 9 ). The small travel time difference between the primary and ghosts could introduce notches into the spectra of the seismic data, reducing the bandwidth of the signal ( Supplementary Fig. 9f ). The effect of ghost in reducing the low frequency energy plays an important role in imaging very deep structures. Since we know the depth of the streamer and source, and assuming a P-wave velocity of 1500, m s −1 in the water, we can predict the arrival time difference of ghost reflection, which will be 0.02 s for the normal incidence. Then we can generate a ghosted signal response of +1, −2, +1 containing both source and receiver ghosts ( Supplementary Fig. 9e ). Corresponding to this ghosted response, the first ghost notch occurs at 50 Hz in the frequency domain. With this information, we can design an inverse filter and remove the effect of the ghosts. From the convolution theory, we calculate the reciprocals of the ghost signal spectrum as an inverse filter. To make it a band limited minimum phase filter, we added a stability factor to the amplitude spectrum, which avoids the minus infinity caused by the alternative Hilbert transform approach and inaccurate signal [60] . By using the synthetic ghosts as input ( Supplementary Fig. 9e ), we filter it with our inverse filter, and obtain a deghosted signal ( Supplementary Fig. 9g ). The amplitude spectrum of input and output ( Supplementary Fig. 9h ) are shown in the units of dB, which indicate that the signal between 0 and 25 Hz has been amplified after the application of the deterministic inverse ghost filter. Similarly, useful amplification is achieved between 25–40 Hz. The deterministic inverse ghost filter is followed by the application of a low pass filter with a cut off at 50 Hz. When we apply this technique to the real data from WG3 and compare our results to the results processed by WesternGeco [27] , our method achieve better performance both in the shallow and the deep parts of the section ( Supplementary Fig. 10 ). Data processing In order to enhance low frequencies and to preserve high frequencies, the pre-stack processing was done in shot, common depth-point (CDP) as well as common receiver domains. The main steps in the shot domain include the removal of the instrument noise caused by the recording instrument anti-alias filter, low frequency enhancement using the deterministic inverse ghost filter, swell noise attenuation and short period multiple attenuation with predictive deconvolution to remove the interlayer multiples. Since the seismic source was powerful, the multiples are very strong and quite challenging to remove. Considering the seafloor reflections arrive at ∼ 6 s two-way-travel time (TWTT), the first multiples will arrive at ∼ 12 s. Furthermore, the raw shot record also contains strong residual shot noise from the previous shot, therefore we used a Radon filter applied to the CDP gathers after parabolic Radon transformation and followed by a tau-p filter after slant-stack transformation in the common receiver gather domain. To preserve primary amplitudes, the demultiple strategy must be oriented to the utilization of the strengths of each methods by combining different methods. The amplitude versus offset analysis is an important tool in demultiple processing. For example, when there is sufficient move-out differential between primaries and multiples, a properly designed Radon demultiple can lead to an effective removal of multiples while preserving primary reflection amplitudes well at the far offsets. So through optimal parameterization, we mute the near offset data in the CDP domain then stack; in this way the primary reflections are preserved with weak residual multiples. Scattering noise reduction was done prior to doing velocity analysis. The last two steps of the processing sequence were CDP stacking and the application of a 2-D time-space post-stack Kirchhoff migration. As shown in Supplementary Fig. 1 , the multiples have been attenuated very well. However, there are some weak flat reflections between 12–16 s, which we interpret as residual multiples. To reduce the uncertainties in the depth conversion, our interval velocity for depth conversion was produced by combining two models from two sources: the part above the Moho came from tomographic inversion results [23] , and the deep part beneath the Moho came from the study of the NoMelt experiment [24] . Relative amplitude calculation Calculating the absolute reflector amplitude of a deep mantle reflector is difficult because the true amplitude gets modified during the data processing. One way to estimate the relative amplitude is to find a shallower continuous reflector that has a good impedance contrast from an interface as a reference reflector and then compute the relative amplitude for the target reflector. Since the Moho reflector here above DMR1 is complex and its amplitude varies along the profile, we decided to use the seafloor amplitude as the reference interface, which is more or less constant along the whole profile. We firstly used a moving window along the DMR1 and DMR2 in the migration image and detected the maximum amplitudes at different depths. We then applied geometric spreading compensation and corrected for the loss of amplitude due to the attenuation as a function of depth. The amplitude ratios for DMR1and DMR2 are shown in Fig. 7a and Supplementary Fig. 8 . Reflection coefficient estimation Normally, we use the seafloor reflection coefficient to estimate the relative reflection coefficient of deep events. Since there are thick sediments, one must take reflection coefficients at each sediment interface into account up to the deep reflector. Since we did not have any constrains on the sediment reflectivity, we used the Moho reflection coefficient as a reference as there were not many reflections between the Moho and the mantle reflectors. We assumed a P wave velocity of 6.8 km s −1 and 7.5–8.0 km s −1 , and the densities to be 2.9 g cm −3 and 3.0–3.1 g cm −3 , above and below the Moho, respectively. Considering the incidence angle at this depth ( ∼ 15 km) is close to zero because of the acquisition geometry, we estimated the reflection coefficient as which gives a Moho reflection coefficient between 0.066 and 0.114. Before calculating the relative amplitude for DMR1 to the Moho, the amplitude of DMR1 should be compensated for relative geometric spreading and Q attenuation, similar to the relative amplitude. The geometric spreading is proportional to the distance, and the material intrinsic attenuation effects can be corrected based on where A 0 is the original amplitude before attenuation, A is the observed amplitude, f is the frequency of the seismic wave, t is the travel time in the medium. Here we assigned Q =1,000 in the mantle for P wave. After correction, we obtained a relative amplitude of ∼ 0.0269 at 16 km depth and ∼ 0.018 at 45 km for DMR1. The amplitude of the Moho is ∼ 0.09, therefore the reflection coefficient values for DMR1 at 16 km would between 0.021 and 0.039, and that at 45 km would be 0.014 and 0.026. These results are consistent with the P wave reflection coefficients that were found for a mantle fault zone in a previous study [61] . Temperature In order to relate our results with the rheology of the lithosphere, we estimated the temperature using the half-space plate-cooling model [62] : where x is the distance from the ridge and z is the depth below the seafloor, a is the asymptotic thermal plate thickness, T m is the basal temperature, and R is the Peclet number relating the advective and conductive heat transfer, v is the half spreading rate, and κ = k /( ρ m C p ) is the thermal diffusivity where k is the thermal conductivity, ρ m is the mantle density and C p is the specific heat. This model is consistent with the model proposed by McKenzie et al . [30] We have used the following parameters [30] , [62] : a plate thickness of 125 km with a basal temperature of 1,350 °C, a coefficient of thermal expansion of 3.28 × 10 −5 K −1 , a specific heat of 1.2 kJ kg −1 K −1 , a mantle density of 3.4 g cm −3 , and a thermal conductivity of 3.14 W m −1 K −1 . We calculated a 2D temperature profile as a function of age and depth. Since the age of the lithosphere along our profile is 55–58 Ma, we plotted one-dimensional temperature along with depth in Figs 7 and 8 . Differential stress estimation The age of the lithosphere in our study area is about 55–60 Ma and the oceanic lithosphere thickness is ∼ 60 km. Though there is no direct way to estimate the strength of the lithosphere, the Byerlee law [63] describes the depth of transition from a brittle, frictional rheology to a temperature-dependent power-law rheology, which can provide some idea of the brittle-plastic transition. For dry olivine, we used the following equation [64] where is the strain rate, A is a pre-exponential factor, σ is the differential stress, n is the stress exponent, Q is the apparent activation energy, R is a constant and T is the absolute temperature. The following parameters were used for dry olivine: A =2.4 × 10 5 s −1 MPa −1 , Q =540 kJ mo1 −1 , n =3.5, R =8.3144 × 10 −3 (refs 46 , 65 ). The geotherm for this area is based on the results from the above temperature calculation. The strain rate is 10 −15 s −1 , the friction coefficient is 0.85 for the Byerlee law. According to a previous study [54] , once the degree of serpentinization reaches ∼ 13%, its effects on rheology will be similar to the rheology of a pure serpentine. Based on the above serpentinization estimation, we have used the lizardite serpentine friction law [65] for the upper 15–25 km, assuming a friction coefficient of 0.3 (ref. 46 , Fig. 7d ). Dip angle of the faults According to the geometrical relationship between the direction of the profile and a true dip along a profile, we can use their dihedral angle and the apparent dip of the two deepest faults to investigate the possible true oblique dip. Since the velocity model estimated from the seismic data dip move-out is not accurate, especially for deep structures, due to the limited offset range of the data, we constructed a time-to-depth conversion velocity model that is made up of two parts. The velocity model for the shallow section above the Moho is derived from travel time tomography. In the mantle, besides Lizarralde et al . velocity model [24] , we also used two other constant velocity models as extreme members for the dip calculation: 7.5 km s −1 and 8.9 km s −1 , respectively. We estimated the dip by projecting these reflectors in different plausible directions of faults ( Supplementary Figs 5 and 6 ). Here we defined the apparent dip as an angle between the horizontal and the tangent line of the dipping mantle reflectors at different depths. The dominant apparent dip of DMR1 on this profile decreases with increasing depth from 40° below the Moho to 12° at ∼ 45 km depth based on the Lizarralde et al . velocity model (ref. 24 , Supplementary Fig. 5a ) and with a ±4° variation ( Supplementary Fig. 5b,c ). As shown in Supplementary Fig. 5 , the projections onto the F5 plane (light blue) have the steepest dip. The dip angles decrease from 50° to 20° with increasing depth when the mantle velocity is 8.9 km s −1 ( Supplementary Fig. 5b ); while they decrease from 45° to 18° for a mantle velocity of 7.5 km s −1 ( Supplementary Fig. 5b,c ). The depth difference of the DMR1 between the lowest and highest velocity is almost 6 km ( Supplementary Fig. 5b,c ). The similar projections for DMR2 are shown in Supplementary Fig. 6 . The DMR2 is steeper than the DMR1 and the dip angle does not change too much with increasing depth. Using the Lizarralde et al . velocity model (ref. 24 , Supplementary Fig. 6a ), the apparent dip of the DMR2 (dark blue) decreases from 30° to 25° from top to bottom, the steepest dip projection is on F6 plane, decreases from 41° to 34°. When we change the velocity model to be a constant mantle velocity of 8.9 km s −1 ( Supplementary Fig. 6b ), the apparent dip of the fault decreases from 35° to 28° from top to bottom, the steepest dip projection on F6 plane decreases from 44° to 36°. The apparent dip of the fault decreases from 28° to 24° when the mantle velocity is 7.5 km s −1 ( Supplementary Fig. 6c ), the steepest dip projection on F6 plane decreases from 40° to 33°. How to cite this article: Qin, Y. & Singh, S. C. Seismic evidence of a two-layer lithospheric deformation in the Indian Ocean. Nat. Commun . 6:8298 doi: 10.1038/ncomms9298 (2015).